Stray-field imaging of magnetic vortices with a single diamond spin Despite decades of advances in magnetic imaging, obtaining direct, quantitative information with nanometre scale spatial resolution remains an outstanding challenge. Recently, a technique has emerged that employs a single nitrogen-vacancy defect in diamond as an atomic-size magnetometer, which promises significant advances. However, the effectiveness of the technique when applied to magnetic nanostructures remains to be demonstrated. Here we use a scanning nitrogen-vacancy magnetometer to image a magnetic vortex, which is one of the most iconic objects of nanomagnetism, owing to the small size (~10 nm) of the vortex core. We report three-dimensional, vectorial and quantitative measurements of the stray magnetic field emitted by a vortex in a ferromagnetic square dot, including the detection of the vortex core. We find excellent agreement with micromagnetic simulations, both for regular vortex structures and for higher-order magnetization states. These experiments establish scanning nitrogen-vacancy magnetometry as a practical and unique tool for fundamental studies in nanomagnetism. Although a remarkable number of magnetic microscopy techniques have been developed over the last decades, imaging magnetism at the nanoscale remains a challenging task because it requires a combination of high spatial resolution and sensitivity [1] . A first approach consists in directly mapping the sample magnetization, which implies sending and collecting back test particles whose interaction with matter has a magnetization-dependent term. This approach provides the highest spatial resolution to date, down to the atomic scale for spin-polarized scanning tunnelling microscopy [2] and about 10 nm in transmission X-ray microscopy [3] . However, these techniques require highly complex experimental apparatus and a dedicated sample preparation so that the particles can reach and escape from the tested region without perturbations. To observe magnetic samples in their real, unprepared state, a more suited approach consists in mapping the magnetic stray field generated outside the sample, even if this method cannot uniquely determine the actual sample magnetization [4] . Furthermore, the spatial resolution is then limited both by the probe size and its distance to the sample. Among many stray-field microscopy techniques [5] , magnetic force microscopy has become ubiquitous, as it provides a spatial resolution <50 nm and operates under ambient conditions without any specific sample preparation [6] . It was for instance the first method that allowed the observation of the core of a magnetic vortex in a thin ferromagnetic disk [7] . However, because of the intrinsic magnetic nature of the probe, magnetic force microscopy is known to be perturbative and not easily quantitative [8] , therefore limiting its field of applications. Recently, a magnetometer based on the magnetic response of a single nitrogen-vacancy (NV) defect in diamond has been proposed [9] , [10] , [11] , [12] , which promises significant advances in magnetic imaging. Indeed, it provides non-perturbing and quantitative measurements of the stray magnetic field, with an unprecedented access to low fields combined with an atomic-sized detection volume [13] , [14] . In this article, we use NV-based magnetometry to measure the stray field emanating from magnetic vortices in nanostructured ferromagnetic thin films. Such structures, which are of great interest both for fundamental studies in nanomagnetism [15] and for applications such as non-volatile magnetic storage [16] , [17] and microwave (MW) generation [18] , have been investigated using a wide range of microscopy techniques [2] , [7] , [19] , [20] , [21] , [22] . However, obtaining quantitative information that is directly comparable to theory remains a challenging task. Further, imaging the vortex core, which can be as small as 10 nm and has a crucial role in the vortex dynamics, is a long-standing goal that has been reached by very few methods only [2] , [3] , [7] . Here we show that scanning NV magnetometry enables to quantitatively map the stray field above a thin ferromagnetic square in a vortex state, revealing in three dimensions the full structure of the magnetic field distribution, including the detection of the vortex core. Furthermore, we demonstrate that the vectorial and quantitative nature of the measurement provide direct comparisons with micromagnetic simulations. This work thus opens new avenues for fundamental studies in nanomagnetism and spintronics. Principle of scanning NV magnetometry The scanning NV magnetometer combines an optical confocal microscope and an atomic force microscope (AFM), all operating under ambient conditions (see Methods). As sketched in Fig. 1a , a diamond nanocrystal hosting a single NV defect is grafted at the apex of the AFM tip and used as an atomic-sized magnetic sensor [13] . The NV defect ground state is a spin triplet with a zero-field splitting D =2.87 GHz between a singlet state m s =0 and a doublet m s =±1, where m s denotes the spin projection along the intrinsic quantization axis of the NV defect u NV ( Fig. 1a ). Under optical illumination, the NV defect is efficiently polarized into the m s =0 spin sublevel and exhibits a spin-dependent photoluminescence (PL) [23] . These combined properties enable the detection of electron spin resonance (ESR) by optical means [24] . A typical ESR spectrum of the NV sensor placed in a static magnetic field is shown in Fig. 1b . In the limit of weak magnetic fields (<3 mT), the spin quantization axis remains fixed by the NV defect axis, and the two ESR frequencies are given by ν R = D ± γ e B NV /2 π , where B NV is the magnetic field projection along the NV axis and γ e is the electron gyromagnetic ratio ( Fig. 1b ). Note that strain-induced splitting of the m s =±1 spin sublevels has been omitted for clarity purpose (see Supplementary Note 1 and Supplementary Fig. S1 ). Measurement of the magnetic field through Zeeman shifts of the ESR frequency is therefore quantitative and non-perturbing, because the dipolar field from a single NV defect is as low as 1 μT at 10 nm distance [9] . 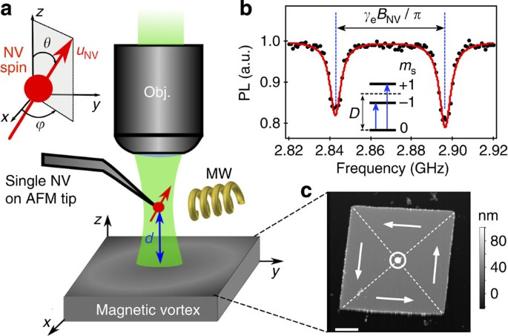Figure 1: Principle of the experiment. (a) The apex of an AFM tip is functionalized with a 20-nm diamond nanocrystal hosting a single NV defect. A microscope objective placed on top of the AFM tip is used both for exciting and collecting the NV defect spin-dependent PL. A MW field is generated by an antenna approached in the vicinity of the NV defect. The NV defect quantization axisuNV, which gives the measured magnetic field component, is described by the anglesθandφin a spherical coordinate system. (b) ESR spectrum of the magnetic probe recorded by monitoring the NV defect PL intensity while sweeping the frequency of the MW field. The ESR splitting is proportional to the projection of the magnetic field along the NV axis, hereBNV=0.9 mT. (c) Typical AFM image of a thin square of Fe20Ni80. The white arrows indicate the curling magnetization of the vortex state. Scale bar, 1 μm. Figure 1: Principle of the experiment. ( a ) The apex of an AFM tip is functionalized with a 20-nm diamond nanocrystal hosting a single NV defect. A microscope objective placed on top of the AFM tip is used both for exciting and collecting the NV defect spin-dependent PL. A MW field is generated by an antenna approached in the vicinity of the NV defect. The NV defect quantization axis u NV , which gives the measured magnetic field component, is described by the angles θ and φ in a spherical coordinate system. ( b ) ESR spectrum of the magnetic probe recorded by monitoring the NV defect PL intensity while sweeping the frequency of the MW field. The ESR splitting is proportional to the projection of the magnetic field along the NV axis, here B NV =0.9 mT. ( c ) Typical AFM image of a thin square of Fe 20 Ni 80 . The white arrows indicate the curling magnetization of the vortex state. Scale bar, 1 μm. Full size image Images of magnetic vortices in ferromagnetic films In the following, we use the scanning NV magnetometer to map the magnetic stray field generated by magnetic vortices in ferromagnetic thin films. More precisely, we investigate squares of Fe 20 Ni 80 with a thickness of 50 nm and a 5-μm side length. This magnetic structure is characterized by a curling in-plane magnetization with a vortex core in the centre where the magnetization points out of the plane ( Fig. 1c ). Such a magnetic vortex is an ideal object for evaluating the sensitivity and spatial resolution of any advanced magnetic microscopy technique because the size of the vortex core can reach 10 nm (ref. 3 ). Furthermore, this magnetic structure is topologically stable and therefore appears as an interesting candidate for memory cells in non-volatile data-storage devices [16] , [17] . The NV probe is first approached at a distance d ≈300 nm above the magnetic vortex structure. Magnetic field mapping is performed by scanning the sample while measuring the difference of NV defect PL intensity for two fixed MW frequencies ν 1 and ν 2 , applied consecutively at each point of the scan [13] . This signal is positive if ν R = ν 1 , that is, when the local field experienced by the NV defect is B NV,1 =±2 π ( ν 1 − D )/ γ e , and negative if ν R = ν 2 , that is, for B NV,2 =±2 π ( ν 2 − D )/ γ e (see Supplementary Methods ). The resulting image thus exhibits positive and negative signal regions corresponding to iso-magnetic field contours ( B NV,1 , B NV,2 ), as well as zero-signal regions for any other field projections. An example of such a dual-iso-B image recorded above a ferromagnetic square is presented in Fig. 2a , revealing a flower-shaped magnetic field distribution. Independent measurement of the NV defect orientation with a calibrated magnetic field indicates that the NV defect is oriented mainly along the y axis in this experiment (see Supplementary Methods and Supplementary Fig. S2 ). Hence, the magnetic map shown in Fig. 2a corresponds to the field component that is parallel to the sample surface and along a side of the ferromagnetic square. By properly selecting the orientation of the single NV defect grafted at the apex of the AFM tip, any field component can be similarly measured. For instance, Fig. 2b is essentially a map of the z component, that is, the out-of-plane magnetic field. These experiments establish NV-based magnetometry as a unique instrument providing quantitative and vectorial magnetic field images at the nanoscale. 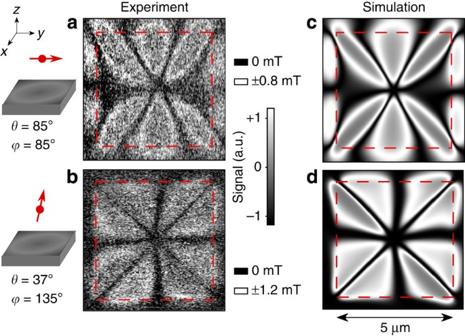Figure 2: Stray-field imaging of a square of Fe20Ni80. (a,b) Dual-iso-B images recorded with a probe-to-sample distanced=400 nm inaandd=300 nm inb. The red squares depict the 5-μm magnetic structure. Ina, the NV is oriented mainly along theyaxis (θ=85°,φ=85°), and inb, the NV defect has a strong component along thezaxis (θ=37°,φ=135°). Images correspond to 200 × 200 pixels, with a 30-nm pixel size and a 60-ms acquisition time per pixel. (c,d) Simulated magnetic field maps corresponding toaandb, respectively. Figure 2: Stray-field imaging of a square of Fe 20 Ni 80 . ( a , b ) Dual-iso-B images recorded with a probe-to-sample distance d =400 nm in a and d =300 nm in b . The red squares depict the 5-μm magnetic structure. In a , the NV is oriented mainly along the y axis ( θ =85°, φ =85°), and in b , the NV defect has a strong component along the z axis ( θ =37°, φ =135°). Images correspond to 200 × 200 pixels, with a 30-nm pixel size and a 60-ms acquisition time per pixel. ( c , d ) Simulated magnetic field maps corresponding to a and b , respectively. Full size image The measured stray field arises from Néel domain walls at the square diagonals that induce volume charges with opposite sign on each side of the wall. The general lobe structure of the magnetic distribution can therefore be qualitatively understood by considering the magnetic field created by an assembly of magnetic dipoles placed along the diagonals. To get more precise predictions, the sample magnetization distribution was first calculated through micromagnetic simulations using OOMMF software [25] , with a cell size of 5 × 5 × 5 nm 3 . Once the equilibrium magnetization state was found, the magnetic field generated by the structure is computed by summing the contribution of all magnetization cells. This magnetic field is then projected along the experimentally measured NV axis, and the NV defect ESR response is finally applied to get the simulated dual-iso-B image (see Supplementary Methods and Supplementary Fig. S3 ). As shown in Fig. 2c,d , the simulations reproduce well the experimental data, including apparent asymmetries which stem from the imperfect alignment of the corresponding NV defects with respect to the y and z axis. By varying the probe-to-sample distance d , it is even possible, as shown in the Supplementary Fig. S4 , to obtain an overview of the stray field in the half-space above the sample, thus providing a three-dimensional mapping of the magnetic field distribution. Imaging the vortex core The magnetic images shown in Fig. 2a,b are recorded with a probe-to-sample distance of several hundreds of nanometres. At such distances, the stray field linked to the out-of-plane vortex core magnetization cannot be detected. The vortex centre therefore appears dark (zero field) both in the images and in the simulations. With the aim of observing the vortex core, the NV probe is brought as close as possible to the sample with the AFM operating in tapping mode. 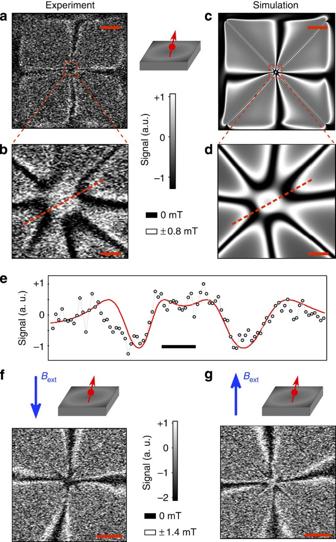Figure 3: Observation of the vortex core. (a) Dual-iso-B image of the whole square obtained with the AFM operating in tapping mode. The same NV probe as inFig. 2bis used (θ=37°,φ=135°). Scale bar, 1 μm. (b) Zoom into the centre of the structure enabling the detection of the stray field emanating from the vortex core magnetization. The image corresponds to 110 × 110 pixels, with a 4.7-nm pixel size and a 60-ms acquisition time per pixel. Scale bar, 100 nm. (c,d) Simulated magnetic field maps corresponding toaandb, respectively, with a probe-to-sample distanced=100 nm. (e) Line-cut taken along the red-dashed line inb(markers) andd(solid line). Scale bar, 50 nm. (f,g) Dual-iso-B image of the square centre while applying a bias field with a projection along the NV axisBext=−0.8 mT infandBext=+0.8 mT ing. Scale bar, 500 nm. Figure 3a shows the dual-iso-B image of the whole square obtained with the NV defect probe used in Fig. 2b , that is, mainly oriented along the z axis. By zooming in the centre of the structure, the vortex core is revealed with an apparent size L core ≈100 nm ( Fig. 3b ). Although the spatial resolution of scanning NV magnetometry is ultimately given by the atomic-sized detection volume, the effective resolving power is rather limited by the probe-to-sample distance, a common feature of any stray-field microscopy technique. Indeed, numerical calculations indicate that the size of the out-of-plane vortex core magnetization is around 20 nm at the sample surface. The probe-to-sample distance can be estimated by comparing the experimental results to magnetic images simulated at different distances from the sample surface. As shown in Fig. 3c–e , a good agreement is obtained for a distance d ≈100 nm. We attribute this relatively large value to an imperfect positioning of the diamond nanocrystal at the apex of the AFM tip. A more precise control of the NV magnetic sensor position could be achieved by using diamond nanopillar probes [14] . Although the simulation fairly agrees with experimental data, we note that the sharp structures lying along the square diagonals ( Fig. 3c ) are not observed in the experimental images ( Fig. 3a ). In those regions, the stray field generated by Néel domain walls is strong enough to induce a mixing of the NV defect electron spin sublevels, which results in an overall reduction of ESR contrast [26] (see Supplementary Note 2 and Supplementary Fig. S5 ). Figure 3: Observation of the vortex core. ( a ) Dual-iso-B image of the whole square obtained with the AFM operating in tapping mode. The same NV probe as in Fig. 2b is used ( θ =37°, φ =135°). Scale bar, 1 μm. ( b ) Zoom into the centre of the structure enabling the detection of the stray field emanating from the vortex core magnetization. The image corresponds to 110 × 110 pixels, with a 4.7-nm pixel size and a 60-ms acquisition time per pixel. Scale bar, 100 nm. ( c , d ) Simulated magnetic field maps corresponding to a and b , respectively, with a probe-to-sample distance d =100 nm. ( e ) Line-cut taken along the red-dashed line in b (markers) and d (solid line). Scale bar, 50 nm. ( f , g ) Dual-iso-B image of the square centre while applying a bias field with a projection along the NV axis B ext =−0.8 mT in f and B ext =+0.8 mT in g . Scale bar, 500 nm. Full size image Chirality and polarity of the vortex state The vortex structure is commonly characterized by two independent binary properties. The chirality c determines whether the in-plane magnetization is curling clockwise ( c =+1) or counterclockwise ( c =−1), whereas the polarity p of the vortex indicates the upward ( p =+1) or downward ( p =−1) magnetization of the core. The apparent pairing of the zero-field contours around the vortex core observed in Fig. 3b directly enables us to determine that c × p =+1 (see Supplementary Note 3 and Supplementary Fig. S6 ). We note that only an absolute value of the field is measured, preventing a direct measurement of the core polarity without additional measurements. This limitation could be overcome by addressing selectively one of the two ESR transitions through circularly polarized MW excitation [27] . Here we gain further insights into the vortex structure by applying an external bias magnetic field along the z axis with a projection B ext along the NV axis. The amplitude of this external magnetic field is chosen weak enough to avoid modifying the sample magnetization, so that B ext just adds up to the regular stray field of the vortex structure. Figure 3f,g shows magnetic images obtained with B ext =−0.8 mT and B ext =+0.8 mT, respectively. The stray field of the vortex core turns dark—the net magnetic field vanishes—with the negative bias field, which reveals that the vortex core magnetization points upward p =+1, and indicates a stray field emanating from the core B core ≈+0.8 mT. Conversely, the core field is increased with a positive bias field because it adds up to B core . From this polarity measurement, the chirality c =+1 can finally be deduced, leading to a full characterization of the vortex structure. Imaging higher-order magnetization distribution As a final experiment, we study a higher-order magnetization distribution on a Fe 20 Ni 80 square dot. As shown in Fig. 4a , highly non trivial magnetic field distributions are observed above some square ferromagnetic structures of the sample. Obviously, these particular squares are not in the regular vortex distribution studied previously. One way to determine the magnetization distribution is to make an assumption about it, compute the expected dual-iso-B image and compare with experimental data. Here the four near-symmetry points distributed around the square centre suggest a magnetization state comprising four vortices distributed around one anti-vortex at the centre ( Fig. 4b ), which is a known equilibrium state in such ferromagnetic structures [28] . Comparison between the simulated ( Fig. 4c ) and measured magnetic images unambiguously validates our hypothesis that this particular square exhibits a four-vortex-one-anti-vortex magnetization state. (Higher-energy magnetization states might have appeared during the sample growth. We verified that applying a strong rotating magnetic field restored all ferromagnetic squares in their minimum-energy single-vortex state.) 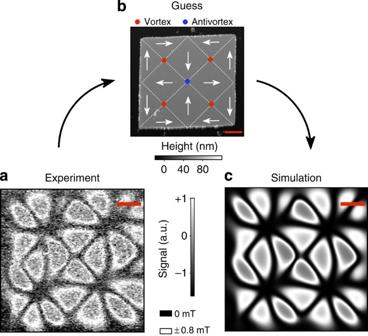Figure 4: Higher-order magnetization distribution. (a) Magnetic field distribution recorded above a square of Fe20Ni80for a probe-to-sample distanced=300 nm. The NV defect orientation is given byθ=65° andφ=30°. (b) AFM image of the square of Fe20Ni80. The white arrows depict the higher-energy magnetization structure, with four magnetic vortices (red dots) distributed around one anti-vortex at the centre (blue dot). (c) Simulated image considering a magnetization following the structure shown inb. Scale bar, 1 μm. Figure 4: Higher-order magnetization distribution. ( a ) Magnetic field distribution recorded above a square of Fe 20 Ni 80 for a probe-to-sample distance d =300 nm. The NV defect orientation is given by θ =65° and φ =30°. ( b ) AFM image of the square of Fe 20 Ni 80 . The white arrows depict the higher-energy magnetization structure, with four magnetic vortices (red dots) distributed around one anti-vortex at the centre (blue dot). ( c ) Simulated image considering a magnetization following the structure shown in b . Scale bar, 1 μm. Full size image These experiments illustrate that scanning NV magnetometry enables robust comparisons with micromagnetic simulations and therefore appears as a powerful tool for fundamental studies in nanomagnetism and, more generally, nanoscience. Indeed, the direct measurement of weak magnetic fields, without perturbation and with a nanoscale resolution, may allow clearing some important issues, such as the nature of magnetic domain walls in ultrathin films with perpendicular anisotropy, which controls their current-induced motion [29] . Bloch- and Néel-type domain walls exhibit distinct stray-field distributions that could be discriminated by scanning NV magnetometry. As an example, micromagnetic simulations indicate that the typical stray field 50 nm above a Bloch wall in a 0.6-nm Co-film with perpendicular anisotropy is ≈5 mT, which changes by ±0.5 mT for a Néel wall (see Supplementary Fig. S7 ). Such a difference is large enough to allow NV magnetometry to experimentally determine the nature of the domain wall and analyse the relevance of Dzyaloshinskii–Moriya interactions in ultrathin magnetic films in contact with non magnetic layers [30] , which is expected to stabilize domain wall into the Néel configuration [31] . The detection of exotic magnetic structures known as skyrmion lattices [32] is another example of a challenge that may be met by scanning NV magnetometry. On a broader perspective, the observation of the stray fields created by persistent currents in micro- and nanostructures where the phase coherence of the carriers is preserved, a quantum realization of the naive Amperian currents proposed two centuries ago to explain the magnetism of matter, appears also within reach of scanning NV magnetometry. Experimental setup and sample fabrication The experimental setup combines a tuning-fork-based AFM and a confocal optical microscope (attoAFM/CFM; Attocube Systems), all operating under ambient conditions. A detailed description of the setup as well as the method to graft a diamond nanocrystal at the apex of the AFM tip can be found in Rondin et al . [13] We use commercially available diamond nanocrystals (SYP 0.05; Van Moppes SA, Geneva), in which single NV defects were created through high-energy electron irradiation (13.6 MeV) followed by thermal annealing at 800 °C. The irradiated nanocrystals were finally oxidized in air at 550 °C during 2 h. This procedure enables to reduce the size of the nanodiamonds and leads to an efficient charge state conversion of the created NV defects into the negatively charged state [33] . For the experiments reported in the main article, the size of the nanodiamonds were in the ~20-nm range, as verified using AFM images before grafting the nanodiamond at the apex of the tip. The unicity of the NV defect was checked through measurements of antibunching in the second-order correlation function g 2 ( τ ) of the NV defect PL, using a standard Hanbury Brown and Twiss interferometer. For ESR spectroscopy, a MW excitation is applied through a 20-μm copper wire directly spanned on the magnetic sample. The 5 × 5 μm 2 square dots were patterned on a silicon substrate using electron-beam lithography followed by evaporation of 50 nm of Fe 20 Ni 80 and lift-off. All experiments were performed at zero external magnetic field, except for the measurement of the vortex core polarity, which required applying a bias field. The acquisition time of all magnetic images was set to 60 ms per pixel corresponding to a total acquisition time of 10 mn for a 100 × 100 pixels image. How to cite this article: Rondin, L. et al . Stray-field imaging of magnetic vortices with a single diamond spin. Nat. Commun. 4:2279 doi: 10.1038/ncomms3279 (2013).